Strong coupling in the sub-wavelength limit using metamaterial nanocavities The interaction between cavity modes and optical transitions leads to new coupled light-matter states in which the energy is periodically exchanged between the matter states and the optical mode. Here we present experimental evidence of optical strong coupling between modes of individual sub-wavelength metamaterial nanocavities and engineered optical transitions in semiconductor heterostructures. We show that this behaviour is generic by extending the results from the mid-infrared (~10 μm) to the near-infrared (~1.5 μm). Using mid-infrared structures, we demonstrate that the light-matter coupling occurs at the single resonator level and with extremely small interaction volumes. We calculate a mode volume of 4.9 × 10 −4 (λ/ n ) 3 from which we infer that only ~2,400 electrons per resonator participate in this energy exchange process. Metamaterials are man-made composites of sub-wavelength building blocks that allow for three-dimensional control of light. Utilization of resonant inclusions allows for the realization of exotic effective medium properties such as negative refractive index [1] , [2] and magnetic response at optical frequencies [3] . This new freedom in design has caused tremendous research interest in recent years. Novel optical designs with stunning properties such as super-resolution [4] , [5] and cloaking [6] have been implemented. Metamaterial resonators may be thought of as highly sub-wavelength electromagnetic cavities, and often exhibit a strong field enhancement in the near-field, making them the ideal candidates for achieving enhanced light-matter interaction. For sufficiently strong interaction, the photon exchange rate between matter and the cavity mode becomes larger than the rates of all the loss mechanisms present in the system. In this case, the electric field radiated by the cavity shows a typical beating mode at a characteristic frequency, called Rabi frequency Ω R . In the frequency domain, this beating corresponds to a splitting of the bare cavity resonance into two polariton branches [7] , [8] , [9] whose energy separation is 2 Ω R . Recently, a new regime called ultra-strong light-matter interaction was demonstrated experimentally in the mid-infrared [10] and terahertz [11] (THz) spectral regions. In this coupling regime the Rabi frequency is comparable to the frequency of the bare cavity resonance. In the description of this system, it is necessary to go beyond the perturbative approach used in standard strong coupling theory by including anti-resonant terms in the interaction Hamiltonian even in equilibrium [12] . To date, all experimental implementations of strong light-matter coupling in the infrared have used wavelength-scale or larger optical cavities such as dielectric microcavities [13] , photonic crystals [14] , planar waveguides [15] , [16] , [17] or gratings [18] , [19] , [20] , [21] . More recently patch antenna arrays including metallic back planes that greatly reduce the interaction volume have been used to demonstrate similar effects [10] . In this work, we demonstrate strong coupling with Rabi splittings on the order of 15% of the fundamental bare cavity frequency in the mid-infrared spectral region using single metamaterial nanocavities with deep sub-wavelength volumes. We show experimentally that the light-matter interaction occurs at the single resonator level. Furthermore, we experimentally demonstrate that this behaviour can be translated to the telecomm spectral range in the near-infrared (~1.5 μm) through appropriate choice of semiconductor materials and metamaterial design. The Rabi splittings demonstrated here are considered to be in the strong coupling limit. We believe that our strategy can be exploited to further increase the Rabi splitting and potentially enter the ultra-strong coupling regime in a near-infrared system that features deep sub-wavelength volumes. Metamaterial nanocavities The basic building block for the work presented here is described schematically in Fig. 1a . It consists of a sub-wavelength ‘dogbone’ [22] metamaterial resonator—the cavity—fabricated directly on top of a ‘dipole’ implemented using optical transitions in a bandgap-engineered semiconductor heterostructure. A scanning electron microscopy image of a fabricated dogbone with a resonance at 31.6 THz is presented in Fig. 1b . We scale the dimensions of this resonator geometry to cover both spectral regions of interest, the mid-infrared (8–12 μm) and the near-infrared (1.5 μm). In the off-resonant case the resonator and the optical dipoles each show a single resonance, as depicted in Fig. 1a . When the two resonances become similar in energy, the two systems couple and the energy oscillates between the electromagnetic field and the optical dipoles. This energy exchange happens at the characteristic Rabi frequency. In contrast to traditional cavity quantum-electrodynamic experiments with atomic systems, neither the matter nor the cavity resonances are ‘sharp’ in the investigations presented here. In fact, both resonances show a typical full-width at half-maximum of 10% of their centre frequencies. Furthermore, all experiments shown here are performed at room temperature as the strong coupling is stable at elevated temperatures. 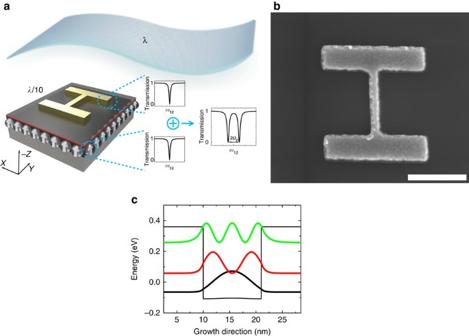Figure 1: Experiment overview. (a) Schematic view of the experiment. The sub-wavelength metamaterial resonator is fabricated on top of a semiconductor substrate. Light illuminates the sample at normal incidence and is polarized along theyaxis. The matter dipoles (ISTs) and the metamaterial resonators show a single resonance. When coupled, the resonance splits into two polariton branches. The plane wave shows the relative length scale of incoming light to metamaterial resonator. (b) Scanning electron microscopy (SEM)-image of a single dogbone-metamaterial resonator with a resonance at 31.6 THz and fabricated using 100 nm thick gold. The scale bar corresponds to 500 nm. (c) Self-consistent band-structure calculation of sample A (λIST: 10 μm). The quantum-well is homogenously doped to a density of 1.25 × 1012cm−2. The optically active transition happens between the ground state (black) and the first excited state (red). The Fermi level is set between these two levels. Figure 1: Experiment overview. ( a ) Schematic view of the experiment. The sub-wavelength metamaterial resonator is fabricated on top of a semiconductor substrate. Light illuminates the sample at normal incidence and is polarized along the y axis. The matter dipoles (ISTs) and the metamaterial resonators show a single resonance. When coupled, the resonance splits into two polariton branches. The plane wave shows the relative length scale of incoming light to metamaterial resonator. ( b ) Scanning electron microscopy (SEM)-image of a single dogbone-metamaterial resonator with a resonance at 31.6 THz and fabricated using 100 nm thick gold. The scale bar corresponds to 500 nm. ( c ) Self-consistent band-structure calculation of sample A (λ IST : 10 μm). The quantum-well is homogenously doped to a density of 1.25 × 10 12 cm −2 . The optically active transition happens between the ground state (black) and the first excited state (red). The Fermi level is set between these two levels. Full size image The optical dipoles in this work are the intersubband transitions (ISTs) of semiconductor heterostructures. Stacks of thin layers of different semiconductors form potential wells (quantum wells) for electrons inside the conduction band. By appropriately doping the wells, optical transitions between quantized electron levels lead to discrete ‘atomic-like’ absorption spectra. A key advantage of ISTs is the ability to scale the transition energies by using different semiconductors and/or changing the quantum-well (QW) geometry. We employ two different material systems to cover the mid- and near-infrared spectral ranges. Our mid-infrared samples are based on InGaAs/AlInAs heterostructures. While scaling the resonant frequencies of the metamaterial nanocavities to the near-infrared is straight forward, the InGaAs/AlInAs system is not amenable to near-infrared ISTs and we must utilize a different semiconductor material set. III-nitride semiconductor systems have a large conduction band offset and enable ISTs at shorter wavelengths. However, achieving ISTs of sufficient quality in the near-infrared for optical emission is very challenging [23] , [24] . Our near-infrared samples are based on high quality AlGaN/AlN heterostructures that produce ISTs at ~1.5 μm. The exact growth sequence for all samples is given in the Methods section. Mid-infrared strong coupling Experimentally, we study our strong light-matter interaction by performing optical transmission experiments at normal incidence. We fabricated a series of metamaterial samples with different resonator sizes, and hence different resonant frequencies, on top of In 0.53 Ga 0.47 As/Al 0.48 In 0.52 As QW samples. The absorption transition can be tuned from 8 to 12 μm (155–100 meV) by appropriate choice of well thickness. A calculated band structure for sample A (10 μm or 120 meV) is presented in Fig. 1c . As the resonant frequency of the metamaterial nanocavity is varied (by size scaling) across the IST resonance, the normal incidence transmission spectra show two polariton branches with clear anti-crossing behaviour. The predicted transmission curves obtained using finite-difference time-domain simulations and the experimentally observed ones for sample A are shown in Fig. 2a,b respectively. The measured anti-crossing curves are shown in more detail in Fig. 2c . In the off-resonance case a distinct transmission minimum associated with the metamaterial nanocavity resonance is observed along with a weaker minimum due to the IST. When the two resonances become similar in energy, the weights of the two minima become comparable. Exactly on resonance, the spectral position of each of the peaks is shifted from its uncoupled position by Ω R /2π=1.74 THz. In this case, it is impossible to assign either minimum to the metamaterial or to the quantum well response. 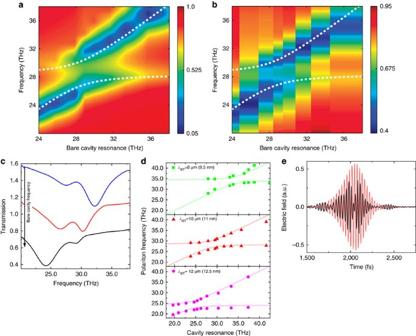Figure 2: Theoretical and experimental polariton anti-crossing curves. (a) Simulated transmission obtained from finite-difference time-domain calculations for sample A (λIST: 10 μm, QW-width: 11 nm). For the simulation, we describe the ISTs as single Lorentzian oscillators37; details are given in the Methods section. The anti-crossing observed between 26 and 34 THz is clearly visible. The dashed, white line shows the quantum-mechanically calculated polariton frequencies. (b) Experimental transmission for sample A (λIST: 10 μm, QW-width: 11 nm). The incoming light is polarized along they-direction. The step-likexaxis indicates that only a discrete number of metamaterial cavities has been fabricated and tested experimentally. (c) Detailed transmission plots for three different metamaterial nanocavities corresponding to bare cavity frequencies of 25.8 (black), 28.9 (red) and 31.6 THz (blue), respectively. The individual curves are offset vertically by 0.35 for clarity. (d) Polariton frequencies for all three mid-infrared samples extracted from transmission spectra. The symbols indicate experimental values; the solid lines are the quantum-mechanical predictions. The figure legend gives the designed IST wavelength, with the width of the quantum-well indicated in brackets. (e) Experimental time trace of Eyfor sample B (λIST: 8 μm, QW-width: 9.5 nm) measure using TDS (black). The beating with a period of 480 fs corresponds to the energy exchange rate between the electromagnetic field and the quantum-wells. The red line represents the incoming pulse. Figure 2: Theoretical and experimental polariton anti-crossing curves. ( a ) Simulated transmission obtained from finite-difference time-domain calculations for sample A (λ IST : 10 μm, QW-width: 11 nm). For the simulation, we describe the ISTs as single Lorentzian oscillators [37] ; details are given in the Methods section. The anti-crossing observed between 26 and 34 THz is clearly visible. The dashed, white line shows the quantum-mechanically calculated polariton frequencies. ( b ) Experimental transmission for sample A (λ IST : 10 μm, QW-width: 11 nm). The incoming light is polarized along the y -direction. The step-like x axis indicates that only a discrete number of metamaterial cavities has been fabricated and tested experimentally. ( c ) Detailed transmission plots for three different metamaterial nanocavities corresponding to bare cavity frequencies of 25.8 (black), 28.9 (red) and 31.6 THz (blue), respectively. The individual curves are offset vertically by 0.35 for clarity. ( d ) Polariton frequencies for all three mid-infrared samples extracted from transmission spectra. The symbols indicate experimental values; the solid lines are the quantum-mechanical predictions. The figure legend gives the designed IST wavelength, with the width of the quantum-well indicated in brackets. ( e ) Experimental time trace of E y for sample B (λ IST : 8 μm, QW-width: 9.5 nm) measure using TDS (black). The beating with a period of 480 fs corresponds to the energy exchange rate between the electromagnetic field and the quantum-wells. The red line represents the incoming pulse. Full size image We demonstrate the ease of spectrally tuning this strong coupling behaviour throughout the mid-infrared by scaling the metamaterial nanocavity dimensions and appropriately varying the IST design. Figure 2d shows the measured and predicted anti-crossing behaviour for three different samples. Starting from sample A with a transition wavelength of 10 μm (QW-width 11 nm), we scaled the resonance to 8 μm (sample B, QW-width 9.5 nm) and 12 μm (sample C, QW-width 12.5 nm), respectively. The anti-crossing frequencies closely correspond to the frequencies of the ISTs for all three samples. The predicted anti-crossing curves were calculated using the theoretical framework described in Supplementary Notes 1 and 3 , which preserves the fermionic character of the electrons and still captures the polaritonic features. This allows us to calculate the line width of the bare IST resonance and the lifetime of the polaritons due to scattering with electrons, phonons and other polaritons (see Supplementary Note 2 and Supplementary Fig. S1 ). We obtain excellent agreement with our theory for all our samples without free fitting parameters for the quantum-mechanical calculations of the polariton branches. The parameters entering the eigenfrequency calculation, such as doping density and the metamaterial resonance frequency, are set during growth and processing. It is interesting to note that the two polariton branches asymptotically approach two different values for large and small bare cavity resonances. The frequency region between the two limiting values is commonly referred to as the ‘polaritonic gap’ [21] , [25] and is estimated to be on the order of 0.2 THz for our samples. Unequivocal demonstration of strong coupling requires the observation of Rabi oscillation in the time domain, in addition to spectral measurements [26] . For this purpose, we performed ultrafast amplitude and phase measurements of the transmitted electric field using time-domain spectroscopy (TDS) in the mid-infrared. Our experimental setup is based on a parametrically amplified, ultrafast fibre laser system seeded by a single ultrashort Er:fibre laser [27] (see Methods). An ultrafast mid-infrared pulse (290 fs full-width at half-maximum), tuned to the anti-crossing frequency, is incident on the sample (sample B, λ IST : 8 μm) and excites the coupled system. The transmitted pulse exhibits a beating behaviour with a period of 480 fs ( Fig. 2e ). This measurement directly confirms the ultrafast energy exchange between the metamaterial nanocavities and the optical dipoles. Furthermore, it shows that we are operating well within the coherence time and the lifetime of the ISTs. The IST in this case (λ IST : 8 μm) shows a broadening of 1.7 THz which corresponds to a lifetime of 600 fs. This value is consistent with previously reported lifetimes for ISTs in In 0.53 Ga 0.47 As/Al 0.48 In 0.52 As QWs in the mid-infrared spectral range [28] . We demonstrate that the strong coupling presented here occurs at a single resonator level of sub-wavelength dimensions (~λ/10) by showing that the same behaviour is observed regardless of the areal density of the metamaterial nanocavities. The results presented thus far were obtained using two-dimensional nanocavity arrays that led to good signal contrast in transmission experiments. To show that the coupling occurs at the single resonator level, we prepared a series of samples containing identical resonators but with an increasing period. The experimental transmission data for the on-resonance case of sample A (λ IST : 10 μm) are shown in Fig. 3a,b . A dilution of one corresponds to the original sample with a period of 2.9 μm. The largest areal dilution fabricated was 100 that corresponds to a resonator spacing of three times the free-space wavelength λ. In our experiments, we use an aperture of 1 mm 2 that translates to 1,200 nanocavities measured simultaneously for the highest areal dilution. The resulting transmission curves show that the splitting energy does not change: only the transmission contrast diminishes with dilution. 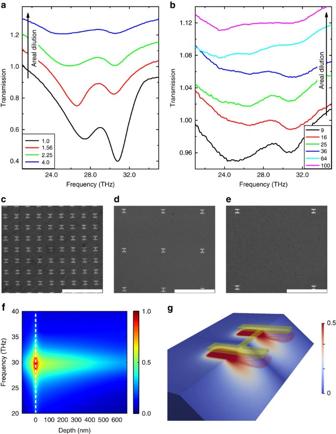Figure 3: Strong coupling occurring at the single resonator level. (a,b) Experimental transmission spectra for different areal dilutions of the metamaterial nanocavities. Panel a shows areal dilutions from 1 (original period of 2.9 μm) to 4, while panel b is from 9 to 100. The splitting remains the same for all dilutions, and only the visibility/contrast is reduced. The aperture size is kept constant at 1 mm2for all dilutions; this corresponds to ~1,200 nanocavities measured at once for the highest dilution. The legends give the exact areal dilution used for each curve. The individual curves are offset vertically for clarity. (c–e) The three SEM images show areal dilutions of 1 (c), 12 (d) and 42 (e). The scale bar corresponds always to 10 μm (the free-space wavelength); the scanned area remains the same in all three images. (f) Calculated spectrally and spatially resolved metamaterial near-fieldEzwithout the quantum-well for sample A. The plottedEzfield is integrated across thexy-plane of the unit cell. The interface air-semiconductor is indicated with the white, dashed line. The electric near-field shows a single resonance and decays away from the metamaterial. (g) Cut through the unit cell of sample A with an areal dilution of 1 showing the absolute value of theEzcomponent on resonance. The electric field remains strongly localized underneath the metallic dogbone resonator indicated by the semi-transparent gold trace. Only the field regions where the value is larger than half the maximum value inside the semiconductor count towards the mode volume. This region is indicated with the red symbols in the figure. Figure 3: Strong coupling occurring at the single resonator level. ( a , b ) Experimental transmission spectra for different areal dilutions of the metamaterial nanocavities. Panel a shows areal dilutions from 1 (original period of 2.9 μm) to 4, while panel b is from 9 to 100. The splitting remains the same for all dilutions, and only the visibility/contrast is reduced. The aperture size is kept constant at 1 mm 2 for all dilutions; this corresponds to ~1,200 nanocavities measured at once for the highest dilution. The legends give the exact areal dilution used for each curve. The individual curves are offset vertically for clarity. ( c – e ) The three SEM images show areal dilutions of 1 ( c ), 12 ( d ) and 42 ( e ). The scale bar corresponds always to 10 μm (the free-space wavelength); the scanned area remains the same in all three images. ( f ) Calculated spectrally and spatially resolved metamaterial near-field E z without the quantum-well for sample A. The plotted E z field is integrated across the xy -plane of the unit cell. The interface air-semiconductor is indicated with the white, dashed line. The electric near-field shows a single resonance and decays away from the metamaterial. ( g ) Cut through the unit cell of sample A with an areal dilution of 1 showing the absolute value of the E z component on resonance. The electric field remains strongly localized underneath the metallic dogbone resonator indicated by the semi-transparent gold trace. Only the field regions where the value is larger than half the maximum value inside the semiconductor count towards the mode volume. This region is indicated with the red symbols in the figure. Full size image The individual resonator origin of the strong coupling, combined with the fast decay of the resonator near fields, implies that the mode coupling volume is extremely small. The frequency and spatially resolved E z -profile of a single dogbone resonator without the influence of the QWs obtained using a finite-difference time-domain calculation is presented in Fig. 3f . The results show the expected single resonance and a rapid decay of E z into the semiconductor region with a typical decay length of a few hundred nanometres. Thus, the QWs have to be grown very close to the surface to interact with the metamaterial resonator. To calculate the interaction volume precisely, we use the full 3D on-resonance E z field distribution shown in Fig. 3g , and only include regions where the absolute value of E z is larger than half of the maximum value inside the quantum-well region. This method avoids the problems due to strong field enhancement at metal surfaces (see Methods for details). With this approach, we estimate an effective volume of ~1.2 × 10 −2 μm 3 (or 4.9 × 10 −4 (λ /n ) 3 ) regardless of the areal dilution. It should be noted that due to the design of our metamaterial nanocavities, a metallic backplane is not required to achieve this efficient modal confinement and to efficiently convert the incident fields to the E z polarization required for excitation of the ISTs. Using a QW doping density of 1.25 × 10 12 cm −2 and QW period of 31 nm, we calculate that only ~2,400 electrons participate in the energy exchange between the IST and the cavity mode on a single resonator level. This allows the study of strong light-matter interactions with an extremely small number of electrons. Near-infrared strong coupling Translating this metamaterial nanocavity-based strong coupling behaviour to shorter wavelengths will allow the exciting properties arising due to extremely efficient energy exchange to be studied using single photon techniques available at near-infrared and shorter wavelengths. We achieve this first step by scaling the metamaterial nanocavities and coupling them with ISTs in the Al 0.03 Ga 0.97 N/AlN system. We exploit the large conduction band offset present in Al 0.03 Ga 0.97 N/AlN heterostructures to tune the IST to 1.52 μm. A self-consistent bandstructure calculation of such a heterostructure is presented in Fig. 4a . A scanning electron micrograph of a scaled dogbone-metamaterial nanocavity is shown in Fig. 4b . 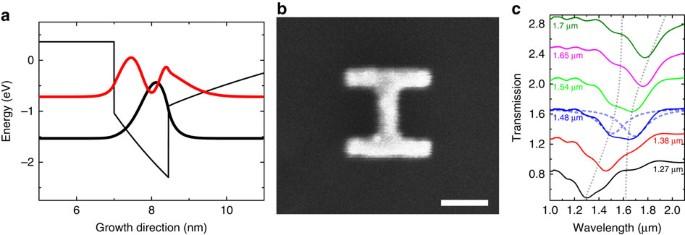Figure 4: Strong coupling at near-infrared wavelengths. (a) A self-consistent band-structure for our Al0.03Ga0.97N/AlN quantum-well using an eight-bandk.pmethod. The black line represents the ground state, the red one the first excited one of the quantum-well. The additional band-bending is caused by the built-in field due to the highly polar nature of the crystal. (b) SEM images for our dogbone resonator designed for the near-infrared. The smallest feature sizes are on the order of 30 nm. The gold film thickness is reduced to 50 nm compared with our mid-infrared samples. The scale bar corresponds to 100 nm. (c) Experimental transmission curves for the near-infrared sample. The polariton splitting for bare cavity resonances around 1.5 μm reaches 10% of the centre frequency. The bare cavity resonance wavelengths are given next to each curve. The individual curves are offset vertically by 0.4 for clarity. The two dashed blue lines show the two minima which are shifted from the natural eigenfrequencies due to the strong light-matter coupling. The dotted grey lines are a guide to the eye illustrating the polariton anti-crossing. Figure 4: Strong coupling at near-infrared wavelengths. ( a ) A self-consistent band-structure for our Al 0.03 Ga 0.97 N/AlN quantum-well using an eight-band k.p method. The black line represents the ground state, the red one the first excited one of the quantum-well. The additional band-bending is caused by the built-in field due to the highly polar nature of the crystal. ( b ) SEM images for our dogbone resonator designed for the near-infrared. The smallest feature sizes are on the order of 30 nm. The gold film thickness is reduced to 50 nm compared with our mid-infrared samples. The scale bar corresponds to 100 nm. ( c ) Experimental transmission curves for the near-infrared sample. The polariton splitting for bare cavity resonances around 1.5 μm reaches 10% of the centre frequency. The bare cavity resonance wavelengths are given next to each curve. The individual curves are offset vertically by 0.4 for clarity. The two dashed blue lines show the two minima which are shifted from the natural eigenfrequencies due to the strong light-matter coupling. The dotted grey lines are a guide to the eye illustrating the polariton anti-crossing. Full size image The optical transmission spectra obtained for different scalings of the dimensions of the metamaterial nanocavities are shown in Fig. 4c . Anti-crossing behaviour is observed in a manner similar to the mid-infrared case, with an on-resonance energy separation of 10% of the bare cavity photon energy. This splitting is somewhat smaller than was obtained in the mid-infrared case. We attribute this to fundamental scaling properties of strongly coupled systems when moving towards shorter wavelength: the ratio of Rabi frequency to bare cavity frequency which determines the visibility of the strong coupling in the experiment scales with the square root of the wavelength [12] . Therefore, for a fixed oscillator strength, the experimental realization of strong coupling is easier at longer wavelengths. For future experiments the interaction can be increased by optimizing the metamaterial nanocavity (for example, reduction of the mode volume) and the QW design (for example, increase of the oscillator strength). It is interesting to note that the smaller mode volume of the near-infrared metamaterial nanocavities is compensated by a larger QW doping density, which leaves the number of electrons participating in the strong coupling per resonator nearly unchanged. We have presented an unambiguous experimental demonstration of strong light-matter interaction using sub-wavelength metamaterial nanocavities throughout the near- and mid-infrared spectral range. We exploit the giant matrix elements of ISTs in semiconductor QWs and couple them to dogbone-metamaterial resonators. We directly measured the energy exchange between the coupled light-matter states in the time domain in the mid-infrared and observed Rabi oscillations with a period of 480 fs. The splitting between the upper and lower polariton branches corresponds to 15% of the centre frequency in the mid-infrared and 10% at near-infrared wavelengths. A system consisting of a single metamaterial nanocavity strongly coupled to optical dipoles in semiconductor heterostructures shows great potential for new studies in the science of light-matter interaction as well as for new optoelectronic device concepts. Using an array of these nanocavities, it is easy to build macroscopic optical filters and modulators at any given wavelength. The IST energy and thus the occurrence of strong coupling can be controlled by the application of a voltage. This tuning strategy is easier to realize than tuning using physical deformation of a metamaterial [29] or conventional permittivity changes by depletion [30] , [31] , [32] and is faster compared with thermal tuning [33] , [34] . From a fundamental science point of view a remarkable feature of our system is that the light-matter interaction occurs on a single resonator level. As a result, the strong coupling is realized with a very small number of electrons (~2,400 per resonator in our case, and this number could be reduced even further), making this an ideal tool to explore many-body effects in a well-defined system with a limited number of contributing carriers. In addition, each coupled metamaterial nanocavity can be understood as a single light emitter which can be positioned freely. Therefore, it would be possible to study the coupling between individual emitters and explore unusual effects such as superradiance [35] . It should be stressed that the nanocavity itself and the spacing between two adjacent nanocavities are sub-wavelength. Furthermore, we have also demonstrated the scaling of this strong light-matter interaction approach to near-infrared wavelengths (1.5 μm) using III-nitrides. The short wavelength regime is highly interesting since it allows the study of photon statistics using readily available experimental techniques. Sample details The mid-infrared samples are based on the In 0.53 Ga 0.47 As/Al 0.48 In 0.52 As material system that is lattice matched to the InP substrate. The near-infrared samples are Al 0.03 Ga 0.97 N/AlN quantum-wells; this sample is grown on a sapphire substrate with a 1.3-μm thick AlN buffer layer. The exact growth sequences including the doping levels are given for all four samples in Table 1 . Table 1 Quantum-well details. Full size table Finite-difference time-domain calculations The finite-difference time-domain simulations are performed using a commercial code (Lumerical, http://www.lumerical.com ). The ISTs are modelled in the numerical finite-difference time-domain simulation as anisotropic Lorentzian oscillators. The permittivity of the entire active region is described as [36] , [37] : where ε InGaAs describes the background permittivity of the QW, N D the carrier concentration, e the electron charge, m * the effective electron mass, f 12 the oscillator strength, the IST including the depolarization shift and δ the broadening of the IST. The gold for the metamaterial is described using a standard Drude model [38] with a plasma frequency of 2,060 THz and a damping of 10.9 THz. These values are extracted from spectral ellipsometry measurements on a 100-nm thin gold film that was evaporated under identical conditions as the metamaterial samples. Time-domain spectroscopy system A schematic of our time-domain spectroscopy system is presented in Fig. 5 . The fibre laser system used in our time-domain spectroscopy measurements produces three parametrically amplified outputs and is seeded by a single ultrashort Er:fibre laser. Two pulse trains are mixed in a GaSe crystal to generate the broadband mid-infrared pulses that can be tuned from 7 to 13 μm. The 15 fs gate pulse is used to measure the mid-infrared transient in a second GaSe crystal using phase-matched electro-optic sampling [39] . The combination of this generation and detection scheme allows us to measure the amplitude and phase of the transmitted or reflected electric field instead of only its intensity. 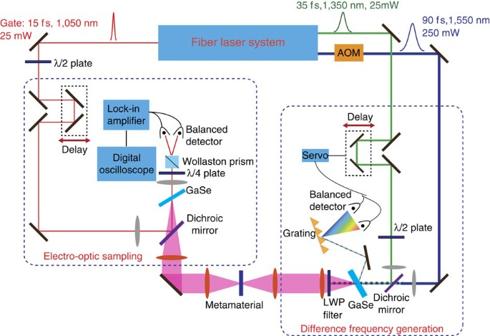Figure 5: Schematic of the mid-infrared TDS system. The carrier-envelope phase is stabilized using the light reflected off the GaSe crystal with a piezo controlled delay feedback loop. Figure 5: Schematic of the mid-infrared TDS system. The carrier-envelope phase is stabilized using the light reflected off the GaSe crystal with a piezo controlled delay feedback loop. Full size image Effective mode volume To calculate our effective cavity mode volume, we use half of the absolute largest E z field value inside the QW-stack as the reference. Only regions where the electric field is larger than half of this reference count towards the mode volume. Using this definition we avoid the problem of extreme field enhancements close to the metal surface and include only the volume coupled to the ISTs. This leads to a mode volume of 1.2 × 10 −2 μm 3 or ~2,400 coupled electrons per resonator given our sheet density of 1.25 × 10 12 cm −2 . If we use the conventional Purcell definition for the effective mode volume of a metamaterial resonator [40] , [41] , [42] , then we would end up with a volume of 10 −3 μm 3 or 4.5 × 10 −5 (λ /n ) 3 . Most of the mode energy of the metamaterial is concentrated within the first few nanometres away from the metal due to the strong field enhancement. However, this part of the mode is not coupled to the ISTs; the closest QW is 30 nm away from the metamaterial. Using this definition for the mode volume would therefore lead to unphysical results for the number of coupled electrons. How to cite this article: Benz, A. et al. Strong coupling in the sub-wavelength limit using metamaterial nanocavities. Nat. Commun. 4:2882 doi: 10.1038/ncomms3882 (2013).